One-by-one trap activation in silicon nanowire transistors Flicker or 1/ f noise in metal-oxide-semiconductor field-effect transistors (MOSFETs) has been identified as the main source of noise at low frequency. It often originates from an ensemble of a huge number of charges becoming trapped and de-trapped. However, as a deviation from the well-known model of 1/ f noise is observed for nanoscale MOSFETs, a new model is required. Here, we report the observation of one-by-one trap activation controlled by the gate voltage in a nanowire MOSFET and propose a new low-frequency-noise theory for nanoscale FETs. We show that the Coulomb repulsion between electronically charged trap sites prevents the activation of several traps simultaneously. This effect induces a noise reduction of more than one order of magnitude. It decreases when the electron density in the channel is increased due to the electrical screening of traps. These findings are technologically useful for any FET with a short and narrow channel. In electronics, noise refers to unwanted or parasitic random signals overlying the useful signals. For most electronics applications, such as amplifiers, memories or digital processing, metal-oxide-semiconductor field-effect transistors (MOSFETs) are the basic constituent of circuits. However, whereas scaling is required for high levels of integration and an increase of working speed, for instance, low-frequency noise is progressively becoming a serious issue for continuous device scaling [1] . Power spectrum current noise in MOSFETs at low frequency follows the 1/ f law, meaning that the noise spectrum is inversely proportional to frequency f on a logarithm scale. The 1/ f noisef is generally interpreted as the superposition of random events of charge trapping and de-trapping from defects randomly distributed in the gate oxide (for example, SiO 2 ) near the semiconductor channel (for example, Si) [2] , [3] ( Fig. 1a ). In shrunk MOSFETs, the number of electrically active defects is reduced, and the low-frequency noise begins to deviate from the 1/ f characteristics [3] , [4] , [5] , [6] . Finally, in submicrometer MOSFETs (for example, <100×100 nm), only a few traps exist, and we observe discrete switching of the drain current between two (or more) levels under constant bias conditions [2] , [3] , [4] , [5] , [6] , [7] , [8] , [9] , [10] ( Fig. 1b ). These fluctuations, known as random telegraph signals (RTSs), give a Lorentzian distribution in the power spectrum current noise. In other words, 1/ f noise, resulting from an averaged ensemble of individual RTSs, is no longer valid in ultrasmall MOSFETs. Therefore, the electrical properties of individual RTS need to be understood to elucidate the noise behaviour in such nanoscale MOSFETs. 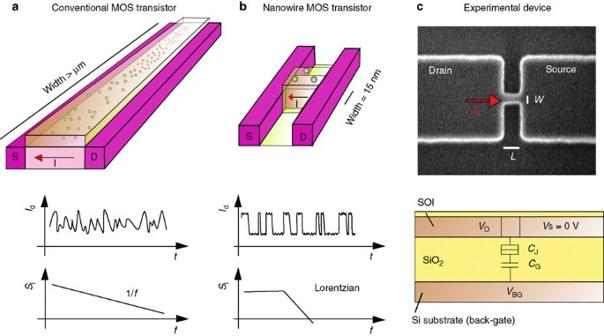Figure 1: General description of trapping/de-trapping noise in transistors. Schematic view of a conventional (a) and nanowire (b) MOS transistor with examples of current fluctuations in the time domain and the corresponding power spectrum noise. Defects are shown as balls and gate oxide with semi-transparent yellow colour. In nano-MOSFETs, fluctuation of the current due to trapping and de-trapping of an electron in a defect leads to discrete steps called random telegraph signals (RTSs) at room temperature and Lorentzian power spectrum noise. Owing to the huge number of traps located at different depths in the oxide in conventional transistors, the 1/flaw is obtained as a sum of Lorentzian spectra with different corner frequencies. (c) Scanning electron microscope image of the Si nanowire and source and drain regions (top view) and schematic side view of an SOI MOSFET with a constriction with dimensionsWandLof 30 and 60 nm, respectively, before thermal oxidation. Scale bar, 200 nm. The oxidation process reduces the size of the constrictionWto about 15 nm (see Methods). To observe the RTS, we chose a MOSFET with few trap sites in the gate oxide surrounding the SOI channel (some MOSFETs show no RTS characteristics due to their small and high-quality channel). The equivalent circuit is given by two capacitorsCGbetween the Si back-gate and the trap site andCJbetween the constricted channel and the trap site. Because the trap site is close to the channel, an electron is trapped there by a tunnelling event through a thin oxide layer. To distinguishCJfromCG, we callCJa tunnelling capacitor and draw it in a way different from conventional capacitorCGas show in the figure. Figure 1: General description of trapping/de-trapping noise in transistors. Schematic view of a conventional ( a ) and nanowire ( b ) MOS transistor with examples of current fluctuations in the time domain and the corresponding power spectrum noise. Defects are shown as balls and gate oxide with semi-transparent yellow colour. In nano-MOSFETs, fluctuation of the current due to trapping and de-trapping of an electron in a defect leads to discrete steps called random telegraph signals (RTSs) at room temperature and Lorentzian power spectrum noise. Owing to the huge number of traps located at different depths in the oxide in conventional transistors, the 1/ f law is obtained as a sum of Lorentzian spectra with different corner frequencies. ( c ) Scanning electron microscope image of the Si nanowire and source and drain regions (top view) and schematic side view of an SOI MOSFET with a constriction with dimensions W and L of 30 and 60 nm, respectively, before thermal oxidation. Scale bar, 200 nm. The oxidation process reduces the size of the constriction W to about 15 nm (see Methods). To observe the RTS, we chose a MOSFET with few trap sites in the gate oxide surrounding the SOI channel (some MOSFETs show no RTS characteristics due to their small and high-quality channel). The equivalent circuit is given by two capacitors C G between the Si back-gate and the trap site and C J between the constricted channel and the trap site. Because the trap site is close to the channel, an electron is trapped there by a tunnelling event through a thin oxide layer. To distinguish C J from C G , we call C J a tunnelling capacitor and draw it in a way different from conventional capacitor C G as show in the figure. Full size image Here, we show that one-by-one activation of RTSs at room temperature can be controlled by the gate voltage of nanoscale MOSFETs. This one-by-one activation is attributed to Coulomb repulsion between electrons trapped in neighbouring defects [5] , [11] , [12] . We establish equations for low-frequency noise in such nanoscale MOSFETs and demonstrate a drastic reduction of this low-frequency noise. Moreover, we show that electrical screening by the electrons in the semiconductor channel reduces this one-by-one activation. Device structure Scanning electron microscope top and schematic side views of the device are shown in Figure 1c . Large undoped silicon-on-insulator (SOI) channels with oxide thickness t ox =400 nm are locally constricted by e-beam lithography and thermally oxidized to form a 40-nm-thick upper oxide (see Methods). The current characteristics are determined by the constricted channel whose width ( W ) and length ( L ) after the oxidation are 15 and 50 nm respectively [13] . The Si substrate is used as the back-gate. Such a small wire channel makes the MOSFET useful as a high-charge-sensitivity electrometer with single-electron resolution [14] , [15] , [16] and thus suitable for a clear observation of RTS at room temperature. Electrons are trapped by oxide defects surrounding the SOI channel at a tunnelling distance (for example, <3 nm) [2] . For a basic equivalent circuit ( Fig. 1c ), we consider the capacitance C G between the gate and trap site and tunnelling capacitance C J between the channel and trap site. RTS amplitude in an Si nanowire transistor Trapping and de-trapping of a single electron by and from a single trap close to the Si channel induce a two-level fluctuation of the drain current called RTS noise due to the electrostatic effect caused by the electron. This RTS noise gives us access to precise information, such as the trap depth (that is, its distance in the oxide from the Si/SiO 2 interface) and gate capacitance C G . In this section, we focus on the analysis of RTS noise amplitude in the nanoscale FETs and, in addition to the aforementioned parameters, we also introduce an effective trap charge, q *, originating from the trapped electron. 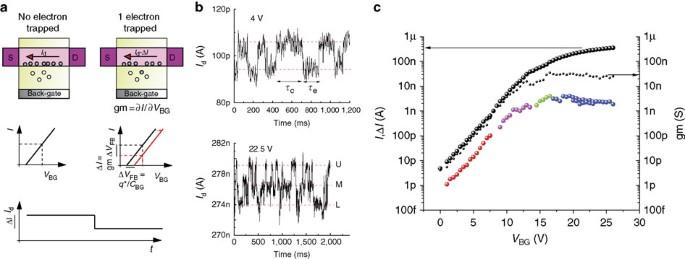Figure 2: Random telegraph signals in an Si nanowire transistors. (a) Schematic description of the impact on drain currentIdof the trapping and de-trapping of an electron in a defect. The two top-sided schematic views of the SiNW transistor show an example of defects without electrons (white balls) and with an electron (one grey ball). SchematicId–VBGcurves for both cases are shown. When an electron is trapped in a defect, it induces a shift of threshold voltage (red curve). At a givenVBG, the current decreases suddenly as shown in the bottom figure. This effect is reversible. (b) Typical RTSs observed in the drain current flowing through a MOSFET atVDof 50 mV and room temperature. Top: Example of two-level RTS atVBGof 4 V. Capture and emission time corresponds to residency time in the upper and lower levels, respectively. Bottom: Three-level RTS atVBGof 22.5 V. U, M and L correspond to the upper, middle and lower levels in the RTS. In both the figures, dotted lines are guides for the eyes for recognition of the two or three levels inId. (c)Id–VBGand gm–VBGcurves are plotted with large and small black circles, respectively. The RTS amplitude ΔI–VBGcurves (coloured circles; trap 1: red, trap 2: purple, trap 3: green, trap 4 and 5: blue) for four traps show almost the same behaviour as gm–VBG. Each RTS coming from its effective trap site is identified as trap 1 to trap 5 from an analysis of the trapping/de-trapping dynamics as shown inFigure 3. Because traps 4 and 5, which give the same ΔI, are active in the same bias range between 20 and 23.5 V (three-level RTS), the number of points is doubled in this range. Figure 2a explains the mechanism of RTS. Let I be the average value of the drain current, I d and Δ I the amplitude of RTS signal. When an electron is trapped by a defect, the electrostatic effect induced by q * shifts current I d as a function of back-gate voltage V BG by Δ V FB . As a result, at a constant gate voltage, this shift corresponds to a small decrease in I d . When an electron is de-trapped from the defect, I d returns to its initial value upon electron de-trapping, thus giving rise to the two-level RTS noise. When C G C J [17] , [18] , simple electrostatics leads to Δ V FB = q*/C G , and from the slope gm=∂ I/ ∂ V BG of the I – V BG curve (gm is the transconductance of the transistor), we get Δ I =gmΔ V FB . Thus, the basic RTS equation is Figure 2: Random telegraph signals in an Si nanowire transistors. ( a ) Schematic description of the impact on drain current I d of the trapping and de-trapping of an electron in a defect. The two top-sided schematic views of the SiNW transistor show an example of defects without electrons (white balls) and with an electron (one grey ball). Schematic Id–V BG curves for both cases are shown. When an electron is trapped in a defect, it induces a shift of threshold voltage (red curve). At a given V BG , the current decreases suddenly as shown in the bottom figure. This effect is reversible. ( b ) Typical RTSs observed in the drain current flowing through a MOSFET at V D of 50 mV and room temperature. Top: Example of two-level RTS at V BG of 4 V. Capture and emission time corresponds to residency time in the upper and lower levels, respectively. Bottom: Three-level RTS at V BG of 22.5 V. U, M and L correspond to the upper, middle and lower levels in the RTS. In both the figures, dotted lines are guides for the eyes for recognition of the two or three levels in I d . ( c ) I d –V BG and gm –V BG curves are plotted with large and small black circles, respectively. The RTS amplitude Δ I–V BG curves (coloured circles; trap 1: red, trap 2: purple, trap 3: green, trap 4 and 5: blue) for four traps show almost the same behaviour as gm– V BG . 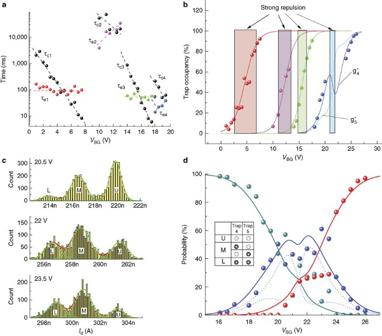Figure 3: Traps occupancy probabilities. (a) Average emission (τei) and capture (τci) interval for trapi(i=1 to 4) as a function ofVBG. (b) Traps occupancy probabilities for five traps. Closed circles are experimental values derived fromτcandτefollowing equation (2) (red: trap 1, purple: trap 2, green: trap 3, blue: trap 4). Solid curves for traps 1–5 are fitted to the experimental values by using equation (3). Shaded areas areVBGranges where strong Coulomb repulsion between electrons located at traps is obtained from equation (4) as plotted inFigure 4b. (c) Histograms ofIdforVBG=20.5, 22 and 23.5 V. (d) Probabilities P(U), P(M) and P(L) of the upper (U), middle (M) and lower (L) levels, respectively, in three-level RTSs plotted as a function ofVBG. Probabilities are obtained by normalizing each peak amplitude. Closed circles are experimental data and solid curves are fitted to experimental results using equations (3) and (4) with parameters shown inTable 1(green: P(U), blue: P(M), red: P(L)). The fit for P(M) can be decomposed into two dashed curves; one for the probability that one electron is trapped at trap 4 and the other that one electron is trapped at trap 5. The inset shows the occupancy status of traps 4 and 5 corresponding to each RTS level. Closed and open circles mean that one or no electron, respectively, is located at the trap site. Each RTS coming from its effective trap site is identified as trap 1 to trap 5 from an analysis of the trapping/de-trapping dynamics as shown in Figure 3 . Because traps 4 and 5, which give the same Δ I , are active in the same bias range between 20 and 23.5 V (three-level RTS), the number of points is doubled in this range. Full size image This equation is widely used for flat band voltage V FB fluctuation [17] as well as for quantifying the behaviour of single-electron memories [14] , [18] . The effective charge q* , which is used instead of the electron unit charge q , depends on V BG and will be discussed later. Basically, we consider q *= q at low gate voltage, that is, in the subthreshold region [19] ( V BG < V FB =12 V here), and q *< q above V FB . Figure 2b shows two examples of RTSs measured in our Si nanowire MOSFET. The upper panel shows basic two-level current fluctuation behaviour, and the lower one shows a more sophisticated three-level current fluctuation, which will be discussed later (see section Coulomb repulsion analysis). Figure 2c shows I–V BG , Δ I–V BG and gm –V BG characteristics. We distinguish the RTS contributions of five traps in the Δ I–V BG curve from a detailed analysis of the time dynamics of the RTS signal (see next section). Then, from the data in Figure 2c (limited below V FB =12 V to assume q *= q ) and from equation (1), we obtain C G =0.91±0.18 aF, which is a realistic value from the viewpoint of device geometry. This proves the validity of equation (1) related to RTS amplitude. Such a clear RTS amplitude dependence of the transconductance gm for several traps is obtained because the oxide thickness between the channel and gate is much larger than the trap depth (distance from the Si nanowire, see Fig. 1c ), that is, C G is much smaller than C J , and because the device dimensions (in particular the width) are much smaller than the Debye screening length (here ∼ 110 nm at room temperature and for an Si nanowire doped at 10 15 cm −3 ); otherwise, the trapped charges in the defects would make the RTS analysis more complicated. As a consequence, such RTS measurement in a nanoscale MOSFET is a highly effective metrology tool for evaluating gate capacitances in the subattofarad range, which is very difficult with other techniques. Trap occupancy probabilities To identify the RTS signal from each trap site, we record the time duration of the high and low currents for a large number of such RTS fluctuations, as shown in Figure 2b . According to the standard statistical analysis [2] , we deduce the average electron capture time ( τ c ) and emission time ( τ e ). Figure 3a shows the V BG dependence of τ c and τ e . We can identify four sets of τ e and τ c at different values of V BG , corresponding to four traps and, more interestingly, can see that the four RTSs become active in turn with increasing V BG . Hereafter, we refer to those sites as traps 1–4 as shown in Figures 2c and 3a . For trap i ( i =1–4), the probability that a trap is occupied by an electron g i = τ e /( τ e + τ c ) also shows a clear one-by-one activation of RTSs. The behaviour of such one-by-one activation of RTSs seems to be unnatural in the well-known RTS theory because it means that trap sites have well-aligned energy levels, although the energy levels are expected to be randomly distributed in space and energy. We will show below that Coulomb repulsion between electrons trapped by a defect can satisfactorily explain this behaviour. Figure 3: Traps occupancy probabilities. ( a ) Average emission ( τ ei ) and capture ( τ c i ) interval for trap i ( i =1 to 4) as a function of V BG . ( b ) Traps occupancy probabilities for five traps. Closed circles are experimental values derived from τ c and τ e following equation (2) (red: trap 1, purple: trap 2, green: trap 3, blue: trap 4). Solid curves for traps 1–5 are fitted to the experimental values by using equation (3). 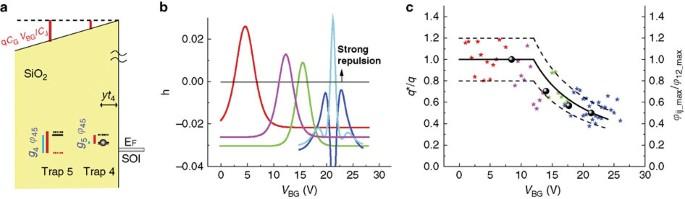Figure 4: Coulomb repulsion and trap effective charge. (a) Energy band diagram of traps 4 and 5. WhenVBGis applied, the potential drop in the oxideCGVBG/CJlowers the trap's energy levels from a dotted black line to a dotted red line. Coulomb repulsion caused by the electrons in trap 4 (trap 5) increases the energy level of trap 5 (trap 4) byg4ϕ45(g5ϕ45) as indicated by a blue line. Therefore, the final energy level of trap sites is raised to the solid black line. (b)hi–VBGcharacteristics given by equation (4).hi>0 means that there is a strong repulsion coming from other traps, that is, only one trap is active at the same time. This repulsion area is reported in traps occupancy probability inFigure 3b. (c) Normalized effective charge obtained by RTS amplitude (closed circles) and normalized Coulomb repulsion potential (closed stars; red: trap 1, purple: trap 2, green: trap 3, blue: traps 4 and 5) withϕ12_max=220 mV as a function ofVBG. The solid curve given by equation (5) fits the experimental results well (withtacc=4 Å andVFB=12 V). Dotted lines are error margins (±20%, corresponding to the accuracy of the determination ofCG) of the fit. Shaded areas are V BG ranges where strong Coulomb repulsion between electrons located at traps is obtained from equation (4) as plotted in Figure 4b . ( c ) Histograms of I d for V BG =20.5, 22 and 23.5 V. ( d ) Probabilities P(U), P(M) and P(L) of the upper (U), middle (M) and lower (L) levels, respectively, in three-level RTSs plotted as a function of V BG . Probabilities are obtained by normalizing each peak amplitude. Closed circles are experimental data and solid curves are fitted to experimental results using equations (3) and (4) with parameters shown in Table 1 (green: P(U), blue: P(M), red: P(L)). The fit for P(M) can be decomposed into two dashed curves; one for the probability that one electron is trapped at trap 4 and the other that one electron is trapped at trap 5. The inset shows the occupancy status of traps 4 and 5 corresponding to each RTS level. Closed and open circles mean that one or no electron, respectively, is located at the trap site. Full size image Coulomb repulsion analysis For the analysis of the Coulomb repulsion, let us return to the three-level RTS observed in the bias range 20.5 V< V BG <23.5 V ( Fig. 2b ). The three-level RTS implies two traps active simultaneously with the same Δ I . This is attributed to trap 4 and another trap (trap 5). Upper (U), middle (M) and lower (L) levels mean that no trap, only one trap and both traps are filled with electrons, respectively. In this bias range, the histograms of the U, M and L levels in I d follow a Gaussian distribution with a relative amplitude that depends on V BG . Figure 3c shows histograms at V BG =20.5, 22 and 23.5 V. Because the amplitudes of the peaks depend on V BG , normalization of each amplitude allows evaluation of probabilities P U , P M and P L of U, M and L levels, respectively, in three-level RTSs ( Fig. 3d ). With g 4 and g 5 as the occupancy probabilities of traps 4 and 5, we get P U =(1− g 4 )( 1 − g 5 ), P M =g 4 ( 1 − g 5 )+ g 5 ( 1 − g 4 ) and P L =g 4 g 5 for the trap conditions illustrated in the inset of Figure 3d . To evaluate P U , P M and P L , we first use the usual g partition function for traps 4 and 5 (g 4 and g 5 ): where E T i is the difference between the trap potential energy ( i =1 to 5) and Fermi energy at V BG =0 V, C J i is C J of trap i , C G the back-gate capacitance (see Fig. 1d ), k the Boltzman constant, T the temperature, q the electron charge and V BG the back-gate voltage. However, equation (2) leads to poor fits ( Supplementary Figure S1 ). To obtain satisfactory fits for P U , P M and P L , we use by introducing an additional term g j ′ ϕ ij (equation 1). The g j ′ ϕ ij corresponds to the Coulomb repulsion potential between trap i and trap j , weighted by occupancy probability g j ′ of the interacting trap j . Using equation (3) instead of equation (2) for the probabilities P U , P M and P L allows us to obtain a reasonable fit as shown in Figure 3d . From this analysis, we can extract occupancy probabilities g 4 ′ and g 5 ′ of traps 4 and 5 as reported in Figure 3b . The qualitative meaning of this modified equation (equation 3) can be simply illustrated with a band energy diagram ( Fig. 4a ) showing how traps 4 and 5 cause the three-level RTS. The key point is a competing effect, quantified by h i , of Coulomb repulsion g j ϕ ij and V BG -induced potential drop C G V BG /C J i of the trap energy level, where h j can be given by Figure 4: Coulomb repulsion and trap effective charge. ( a ) Energy band diagram of traps 4 and 5. When V BG is applied, the potential drop in the oxide C G V BG /C J lowers the trap's energy levels from a dotted black line to a dotted red line. Coulomb repulsion caused by the electrons in trap 4 (trap 5) increases the energy level of trap 5 (trap 4) by g 4 ϕ 45 ( g 5 ϕ 45 ) as indicated by a blue line. Therefore, the final energy level of trap sites is raised to the solid black line. ( b ) h i – V BG characteristics given by equation (4). h i >0 means that there is a strong repulsion coming from other traps, that is, only one trap is active at the same time. This repulsion area is reported in traps occupancy probability in Figure 3b . ( c ) Normalized effective charge obtained by RTS amplitude (closed circles) and normalized Coulomb repulsion potential (closed stars; red: trap 1, purple: trap 2, green: trap 3, blue: traps 4 and 5) with ϕ 12_max =220 mV as a function of V BG . The solid curve given by equation (5) fits the experimental results well (with t acc =4 Å and V FB =12 V). Dotted lines are error margins (±20%, corresponding to the accuracy of the determination of C G ) of the fit. Full size image In the range of V BG between 18 and 23.5 V, the energy level of trap 4 aligns close to that of trap 5, which leads to three-level RTSs. However, as trap 5 is located deeper from the channel than trap 4, as shown in Table 1 (see Methods for the determination of trap depth), removing an electron from trap 5 is harder than removing one from trap 4. More importantly, the Coulomb repulsion is larger than the potential drop of trap sites caused by the applied bias V BGs ; that is, h 5 is positive. Therefore, in this V BG range (18–23.5 V), we can now describe the coupled behaviour of traps 4 and 5 ( Fig. 3b ). As occupancy probability of trap 4 increases with V BG , energy level of trap 5 increases (kink in g 5 ′). Because the rise in the energy level is enough to get complete blockade, occupancy probability of trap 5 increases and pushes up energy level of trap 4 (decrease of g 4 ′). When trap 5 is almost always filled, occupancy probability of trap 4 increases again (increase of g 4 ′). The estimated Coulomb repulsion between traps 4 and 5, ϕ 45 , is 110 meV (see Table 1 ). Table 1 Extracted parameters from RTS. Full size table This Coulomb effect also explains the one-by-one activation of RTSs shown in Figure 3b , that is, the fact that there is no overlap of the occupancy functions of traps 1, 2 and 3. The data are well separated along the V BG axis and equation (3) well reproduces this behaviour. This means that the shaded areas in Figure 3b correspond to high Coulomb repulsion as indicated by the positive values of h j ( Fig. 4b ) for traps 1, 2 and 3. The more complicated curve for V BG >18 V corresponds to the interacting behaviour between traps 4 and 5 as discussed above. As a consequence, it could be concluded that the energy levels of traps when empty are close to each other, which is natural and more feasible given a similar chemical structure. These considerations based on equations (3) and (4) can explain the one-by-one activation of RTSs shown in Figure 3b , that is, no overlap (shaded areas in Fig. 3b ) between each g i ′s at positive h j in particular V BG regions of Figure 4b . This idea can also be explained by an analysis of ϕ ij . From the data shown in Figure 2c , using equation (1) and assuming C G does not depend on V BG ( C G =0.91±0.18 aF, see above), we can calculate the effective charge q * for each trap ( Table 1 ). Because t ox =400 nm and SiNW thickness is 15 nm, the oxide capacitance is much lower than a depletion capacitance in silicon. Therefore C G is independent on V BG . The value of q * decreases with increase in V BG after the channel inversion. Interestingly, the same behaviour is observed for the normalized values of ϕ ij , that is, ϕ ij / ϕ 12 . Figure 4c shows this comparison. These features can be explained by considering the trap's image charge [20] and an electrical screening effect originating from the reduction of charges in the inversion layer of the channel, which allows ϕ ij and q * to be given by (see Methods). where ϵ 1 is the dielectric constant of SiO 2 , r ij the distance between two trap sites and t acc the thickness of the inversion layer of the channel. Figure 4c shows the good agreement between the behaviour of ϕ ij and with t acc and r ij equal to 0.4 and 2 nm respectively. This result means that all traps are located within a few nanometers of each other. Derivation of power spectrum noise equations More interestingly and importantly, the above-detailed analysis of q * and ϕ ij based on Coulomb repulsion provides us a better understanding of low-frequency noise in nanoscale MOSFETs [19] and especially its deviation from the well-known 1/ f noise. We address this noise issue, which can have useful implications for design and simulation of nanoscale MOSFETs. In large devices, with the assumption that 1/ f noise is composed of an ensemble of a large number of RTSs originating from traps randomly distributed in space and potential level, the 1/ f power spectrum current noise S I 1 is given by [17] , [19] where N is the number of active traps. This equation predicts an increase of noise with decreasing device area S , because C G and N (at a given trap density) scale with S . We measured the low-frequency noise at different V BG 's (see Methods). 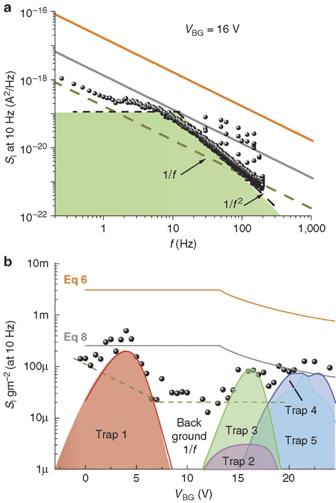Figure 5: Contribution of each trap to power spectrum current noise. (a) ExperimentalSI(closed circles) as a function of frequencyf.SIshows the Lorentzian spectrum, which corresponds to the RTS originating from trap 3 superimposed to a 1/fbackground noise (yellow area). The orange and grey lines are given by equations (6) and (8), respectively. (b) ExperimentalSI/gm2(closed circles) at 10 Hz and comparison with different theories. The bell-shaped curves are given by equation (7), which takes into account the Lorentzian spectrum shape for each trap (filled areas with a different colour for each trap) and equation (8) (grey curve), which is a simplified equation giving an upper limit forSI. A guide for experimental 1/fbackground noise is plotted as a dark dotted line and yellow filling. Note that the shift inVBGfor trap 2 is due to the large time constant for this trap, that is, its Lorentzian corner frequency is10 Hz, which is not the case for other traps. A typical curve measured at V BG =16 V is shown in Figure 5a . The measured noise deviates from strict 1/ f noise and is composed of a 1/ f background noise superimposed by a Lorentzian shape related to the RTS noise generated by trap 3 for this peculiar bias V BG =16 V. An ultimate lower limit of equation (6) calculated for N =1 (one trap, albeit strictly speaking not valid for equation 6) with the gm, q * and C G values for the same V BG (trap 3) clearly overestimates the noise amplitude compared with the experimental data ( Fig. 5a ). When only a few traps are present in nanoscale devices, a better approach is to use the Machlup derivation [2] , [6] , [21] of the Lorentzian equation from RTS. Thus, we can express the low-frequency power spectrum S I 2 i for trap i by (see Methods). Figure 5: Contribution of each trap to power spectrum current noise. ( a ) Experimental S I (closed circles) as a function of frequency f . S I shows the Lorentzian spectrum, which corresponds to the RTS originating from trap 3 superimposed to a 1/ f background noise (yellow area). The orange and grey lines are given by equations (6) and (8), respectively. ( b ) Experimental S I /gm 2 (closed circles) at 10 Hz and comparison with different theories. The bell-shaped curves are given by equation (7), which takes into account the Lorentzian spectrum shape for each trap (filled areas with a different colour for each trap) and equation (8) (grey curve), which is a simplified equation giving an upper limit for S I . A guide for experimental 1/ f background noise is plotted as a dark dotted line and yellow filling. Note that the shift in V BG for trap 2 is due to the large time constant for this trap, that is, its Lorentzian corner frequency is 10 Hz, which is not the case for other traps. Full size image We calculated this quantity at 10 Hz for each trap, i =1 to 5, as a function of V BG using trap parameters ( q *, C G ) and the g i ′ functions in Table 1 and Figure 3b . Each curve is in good agreement with the experimental data. Here τ e i is considered constant with the average value of τ listed in Table 1 . The results are shown as bell-shaped curves and compared with the experimental data in Figure 5b . Each calculated curve is in good agreement with the experimental data. Note that traps 2 and 3 contribute to the noise spectra at 10 Hz for the same range of V BG but with a negligible contribution for trap 2. This is because trap 2 has a higher time constant than trap 3 (see Fig. 3a ). As a consequence, the experimental data around V BG =10 V come from the 1/ f background noise as also observed in Figure 5a . The discussion of the physical origin of this noise is out of the scope of this paper. We suggest elsewhere that it should be due to the dipolar polarization noise in the oxide. For the sake of device simulation, equation (7) is not very practical as it requires a detailed knowledge of the physical parameters of all defects involved in the device. A simplified expression of the maximum of equation (7) can be derived (see Methods) as Equation (8) can be used to estimate the upper limit of noise as shown in Figure 5a,b . Especially, a g i ′ value of 0.5 in equation (7) gives a good estimation of noise SI max at the corner frequency of the Lorentzian spectrum as shown in Figure 5a . This means that when just a few traps are active in nanoscale MOSFETs, the classical equations for 1/ f noise (equation 6) should still be used in device simulation if compensated by a correction factor of about 0.08 as an upper approximation (equation 8). Among the ten measured samples, two did not have any RTS, six had a single RTS and two had many traps (RTSs) with one-by-one trap activation, one of which has been presented here. The second one is shown in Supplementary Figure S2 and an example of single trap is shown in Supplementary Figure S3 . For a high-quality thermal oxide, the typical density of oxide traps is about 10 10 cm −2 in an energy window of kT. These traps are mainly related to dangling bonds in SiO 2 and at the Si/SiO 2 interface [22] . Our device has a surface area of about 15×50 nm and an energy window C G Δ V BG / C Javg =0.7 eV, where C Javg is the average of C J i Table 1 and Δ V BG the window of back-gate voltages. Therefore, the statistical number of traps in our device can be estimated to 2.1, which is not so far from the experimental results from the statistical viewpoint. One-by-one activation of RTSs demonstrated here and the corresponding noise reduction should also be relevant for any other NW-based devices, such as carbon nanotubes and other bottom-up compound semiconductor wires. However, the noise reported is still high [23] , [24] , compared with that state-of-the-art Si MOSFETs. This is because the nanotube in these devices is about 1 μm long, and thus there are many trap sites with no interaction (that is, Coulomb repulsion) between them. Therefore, for the lasting benefit of noise reduction, nanowire devices should have a few-ten-nanometer length, in which Coulomb repulsion between charges located at nearby trapping sites is effective. Farmer et al . [25] have reported the correlation between two RTS events. However, they did not give any detailed analysis for evaluating the RTS amplitude Δ I , the trap occupancy probabilities, the location of trap sites, the Coulomb term ϕ ij , the channel carrier screening effects or the influence on power spectrum noise. We were able to perform such an analysis, because the extremely small gate capacitor of the SOI-based MOSFETs enhances the Coulomb repulsion. Our detailed analysis allows a step-by-step evaluation of the above key parameters of each active trap in a nanoscale FET, and we propose a new model for the low-frequency noise of this nanoscale device suitable for device simulation. Therefore, this nanoscale MOSFET with a short channel and small gate capacitor can be used as a metrological tool for the analysis of capacitances and low-frequency noise. These approaches can be extended as well to devices composed of carbon nanotubes, graphene nanoribbons and any other state-of-the-art nanoscale structures. Device fabrication The nanoscale MOSFETs were fabricated on an SOI wafer. First, a narrow constriction sandwiched between two wider (400-nm wide) channels was patterned on the 30-nm-thick top silicon layer (p-type, boron concentration of 10 15 cm −3 ). The length and width of the constriction channel were 30 and 60 nm, respectively ( Fig. 1c ). The patterning was followed by thermal oxidation at 1000 °C to form a 40-nm-thick SiO 2 layer around the channel. This oxidation process reduced the size of the constriction to about 15 nm, giving a final channel dimension of 15×50 nm. Then, we implanted phosphorous ions outside the constriction, 5 μm away from it, using a resist mask to form highly doped source and drain regions. Finally, aluminium electrodes were evaporated on the source and drain regions. Electrical measurements Electrical measurements were performed at room temperature in a glove-box with a controlled N 2 atmosphere (<1 p.p.m. of O 2 and H 2 O). Drain voltage V D (usually 50 mV) and back gate voltage (<8 V) were applied with an ultralow-noise DC power supply (Shibasoku PA15A1 when V BG <8 V or Yokogawa 7651 when V BG >8 V). The source current was amplified with a DL 1211 current preamplifier supplied with batteries. RTS data and noise spectra were acquired with an Agilent 35670 dynamic signal analyzer (Agilent). Determination of oxide trap depths The trap depths are estimated by fitting with equation (3) the experimental trap occupancy. C J i s obtained for each trap are listed in Table 1 . In a parallel plate configuration, C G i ≈ yt i /t ox , where yt i is the trap depth and t ox is the gate oxide thickness. The t ox =400 nm is larger than width ( W ) and length ( L ) of the nanowire and we cannot neglect border effects. This induces a correction factor of 7.5. Therefore, yt i ≈ C G . t ox /( C J i .7.5) as shown in Table 1 . Theoretical derivation of equation (5) If V BG > V FB , an accumulation layer appears in the Si channel at the SiO 2 interface. This affects the dielectric properties of the Si nanowire. An effective dielectric constant for Si is introduced to consider effects of screening by electrons in the channel. Considering the accumulation charge Q acc related to capacitance C acc , surface potential ψ s , the Debye screening length L d and accumulation layer thickness t acc , we have where W and L are the width and length of the nanowire, C G the back-gate capacitance (see Fig. 1c ), k the Boltzmann constant, T the temperature, q the electron charge, V BG the back-gate voltage, V FB the flat-band voltage, ϵ 0 the vacuum permittivity, ϵ 2 the Si relative dielectric constant, and ϵ 2 ′ the effective Si dielectric constant. From equation (10), we get The electric potential ϕ ij at a distance r ij to the trap and r ij ′ to its image charge [20] is If we consider r ij ≈ r ij ′ (in other words, the distance between traps is large compared to trap depth in oxide), we have Combining equations (11) and (13), we have Then the effective trapped charge q * is given by In this work, the Debye screening length of the undoped silicon is very large ( ≫ 100 nm) compared with the Si thickness (15-nm-thick SOI), so we consider ϵ 2 ≈ ϵ 1 and equation (14) is reduced to equation (5) in the text. Theoretical derivation of equations (7) and (8) We start from the Machlup derivation [21] of power spectrum noise: where Δ I is the RTS amplitude, τ e and τ c the trap emission and capture times, and f the frequency. Considering g = τ e /( τ c + τ e ) and Δ I /gm= q */ C G (see equations 1 and 2), we get At the corner frequency of the Lorentzian distribution, 2 πf (1− g ) τ e =1, and considering g =½, equation (18) becomes How to cite this article: Clément, N. et al . One-by-one trap activation in silicon nanowire transistors. Nat. Commun. 1:92 doi: 10.1038/ncomms1092 (2010).